Unexpected regioselective carbon–hydrogen bond activation/cyclization of indolyl aldehydes or ketones with alkynes to benzo-fused oxindoles Rhodium-catalyzed carbon–hydrogen bond activation has attracted great interest in the construction of carbon–carbon and carbon–heteroatom bonds. In recent years, transition metal-mediated oxygen transposition through a ‘dehydration–rehydration’ process has been considered as a promising strategy towards oxygen-functionalized compounds. Here we describe an unexpected rhodium-catalyzed regioselective carbon–hydrogen bond activation/cyclization of easily available indolyl aldehydes or ketones with alkynes to afford benzo-fused oxindoles, involving the sequential carbonyl-assisted carbon–hydrogen activation of the indole ring at the 4-position, [4+2] cyclization, aromatization via dehydration, nucleophilic addition of water to iminium and oxidation. Isotopic labelling experiments disclose the occurrence of apparent oxygen transposition via dehydration–rehydration from the indolyl-3-carbonyl group to the 2-position of pyrrole to forge a new carbonyl bond. The tandem reaction has been used as the key step for the concise synthesis of priolines, a type of alkaloid isolated from the roots of Salvia prionitis . Rhodium-catalyzed C–H bond activation has attracted great interest in the construction of carbon–carbon and carbon–heteroatom bonds [1] , [2] , [3] , [4] , [5] . In particular, the rhodium-catalyzed coupling reactions of (hetero)aromatic substrates with alkynes have offered a unique platform for atom-economical and straightforward annulation [6] , [7] , [8] , [9] , [10] , [11] , [12] , [13] , [14] . Recently, the research groups of Cheng and co-workers [8] , Glorius and co-workers [9] and Jeganmohan and co-workers [10] have disclosed the synthesis of indenols through the rhodium- or ruthenium-catalyzed carbonyl-assisted aromatic C–H activation/cyclization of aryl ketones with internal alkynes via a proposed five-membered metallocyclic intermediate ( Fig. 1a ). Shi and co-workers [11] have developed the synthesis of indenone by rhodium-catalyzed carbonyl-directed annulation of benzimides with internal alkynes ( Fig. 1b ). Aldehydes often exhibit a poor directing effect and thus examples are still significantly under-represented [15] , [16] , [17] . Usually, ( in situ ) conversion to imines can solve this problem [18] , [19] , [20] . In almost all the previously reported cases, only olefination reactions were studied. 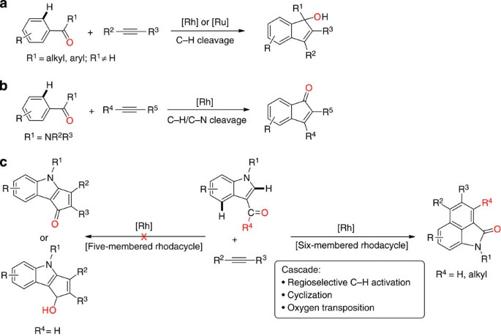Figure 1: Rhodium- or ruthenium-catalyzed carbonyl-assisted (hetero)aromatic C–H activation/cyclization with internal alkynes. (a) In previous work, the preparation of indenols. (b) In previous work, the preparation of indenones. (c) In this report, regioselective carbon–hydrogen bond activation/cyclization to benzo-fused oxindoles. Figure 1: Rhodium- or ruthenium-catalyzed carbonyl-assisted (hetero)aromatic C–H activation/cyclization with internal alkynes. ( a ) In previous work, the preparation of indenols. ( b ) In previous work, the preparation of indenones. ( c ) In this report, regioselective carbon–hydrogen bond activation/cyclization to benzo-fused oxindoles. Full size image (Benzo-fused) oxindoles (indolin-2-ones) are important structural motifs frequently found in pharmaceuticals, natural products and biologically active molecules (for example, antitumor, antibacterial, insecticidal and anthelmintic properties), and are also versatile building blocks for the preparation of structurally complex compounds [21] , [22] , [23] , [24] , [25] . Therefore, the development of new strategies for the facile synthesis of the indolin-2-one scaffolds from easily available starting materials has been an active research area [26] , [27] , [28] , [29] . In an effort to explore the rhodium-catalyzed annulation of indolyl-3-aldehydes with internal alkynes to construct cyclopenta[ b ]indol-1-one or cyclopenta[ b ]indol-1-ol derivatives through the more reactive C2–H cleavage of indole, the benzo-fused oxindoles were obtained unexpectedly through the C4–H activation of indole ( Fig. 1c ) [17] , [30] , [31] , which were confirmed by single crystal X-ray diffraction analysis ( Supplementary Figs 42 and 43 ). This tandem reaction was disclosed to involve an apparent oxygen transposition via dehydration–rehydration from the indolyl-3-carbonyl group to the pyrrole C2-position to forge a new carbonyl bond [32] , [33] , [34] . Based on mechanism investigation, the reactivity and the scope of reaction were further improved. In this work, we would also like to demonstrate the usefulness for the synthesis of natural products. Optimization of the reaction conditions for 3a After we surprisingly observed that the reaction of N -methyl-indolyl-3-carbaldehyde 1a with diphenylacetylene 2a gave benzo-fused oxindole 3a in 39% yield in the presence of 2.5 mol% of [RhCp*Cl 2 ] 2 , 10 mol% of AgSbF 6 and 2.0 equiv. of Ag 2 CO 3 in dioxane at 120 °C for 24 h ( Fig. 2 ; Supplementary Table 1 , entry 1), we started to optimize the reaction system. After screening the different N -substituted indolyl-3-carbaldehydes, N -phenyl-indolyl-3-carbaldehyde 1b afforded 3b in the highest yield of 57% yield ( Supplementary Table 1 , entries 1, 4 and 5). The choice of additive was very crucial for the present catalytic reaction. In the absence of AgSbF 6 , only a trace amount of 3a was obtained ( Supplementary Table 1 , entry 2). Both acids such as PivOH and bases such as CsOPiv could shut down the reactivity ( Supplementary Table 1 , entries 16–17). Other oxidants gave rise to 3b in significantly low yields and even could not deliver the desired product (for example, Cu(OAc) 2 , PhI(OAc) 2 and O 2 ) ( Supplementary Table 1 , entries 12–14). In the absence of Ag 2 CO 3 , the reaction did not occur ( Supplementary Table 1 , entry 15). Tetrahydrofuran (THF) proved to be the best among the solvents investigated ( Supplementary Table 1 , entries 5, 8–11). Increasing loading of [Cp*RhCl 2 ] 2 to 3.5 mol% resulted in a slightly improved yield of 67% ( Supplementary Table 1 , entry 21). 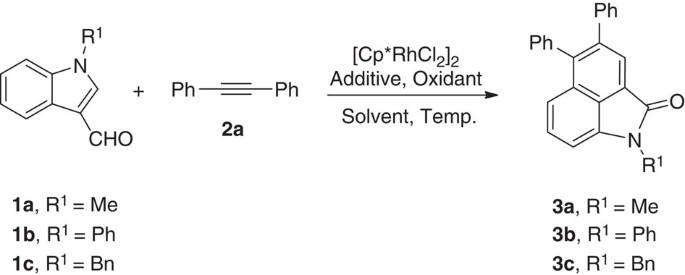Figure 2: Optimization of the Rh-catalyzed tandem reaction of indolyl aldehydes with diphenyl acetylene. See theSupplementary Table 1for details. Figure 2: Optimization of the Rh-catalyzed tandem reaction of indolyl aldehydes with diphenyl acetylene. See the Supplementary Table 1 for details. Full size image Substrate scope With the optimized reaction conditions, the range of indolyl-3-aldehydes was evaluated as illustrated in Table 1 . We were pleased to find that a relatively broad scope of N -substituted indolyl aldehydes could efficiently couple with diphenylacetylene 2a to afford the benzo-fused oxindole derivatives 3 in synthetically useful yields. Both the N -alkyl and N -aryl substituents of indolyl-3-carbaldehydes had little effect on the yields except the N -methyl group ( Table 1 , 3a – 3g ). However, the N -acyl substituted indolyl-3-carbaldehydes could not deliver the desirable product. It is important to stress that the N -benzyl substituted indolyl-3-aldehyde 1c gave rise to 3c in 63% yield, which may further be transformed to the free (NH)-product by removal of the benzyl group. The current catalytic system was tolerant to a variety of synthetically valuable functional groups such as ester, halide and alkyloxyl groups on both the pyrrole ring and the aromatic moiety, which would offer an opportunity for further synthetic transformations. To further expand the scope of the current rhodium catalytic protocol, indolyl-3-ketone was examined as a substrate. However, indolyl-3-ketone exhibited a much lower reactivity than indolyl-3-aldehyde. The coupling reaction of 1-(1-phenyl-1 H -indol-3-yl)propan-1-one 1n with 2a gave 3n in only 30% yield. Table 1 The scope of indolyl-3-aldehydes or ketones. Full size table To test the generality of this protocol, we next examined the scope of internal alkynes. As shown in Table 2 , symmetrical diaryl alkynes, unsymmetrical aryl alkyl alkynes and dialkyl alkynes all could smoothly react with N -phenyl-indole-3-carbaldehydes 1 to afford a variety of benzo-fused oxindoles. Symmetrical diaryl alkynes with both the electron-donating and electron-withdrawing groups could furnish the desired products ( Table 2 , 4a – 4a ). This method was compatible with some important functional groups such as methoxy, fluoro, chloro and bromo groups on the aromatic ring of alkynes. Unsymmetrical aryl alkyl alkynes gave the exclusively regioselective annulation, and the aryl group was installed at the 4-position of benzo-fused oxindole ( Table 2 , 4g – 4i ). Dialkyl alkynes exhibited slightly lower reactivity than diaryl alkynes ( Table 2 , 4j ). Table 2 The scope of alkynes. Full size table Mechanism investigation To probe the plausible mechanism of the cascade reaction, a series of labelling experiments involving 18 O were carried out ( Fig. 3 ; Supplementary Figs 44–48 ). The annulation of 18 O-labelled 1-(1-phenyl-1 H -indol-3-yl)propan-1-one ( 18 O- 1n ) with diphenylacetylene 2a could afford 18 O-labelled benzo-fused oxindole ( 18 O- 3n ), which showed that the oxygen of the carbonyl group in the product originated from the initial material ( Fig. 3a ) [35] , [36] , [37] . Further investigation demonstrated that 18 O could also be incorporated into benzo-fused oxindole 3n when extra 18 O-labelled water was added into the reaction system, which suggested that water might be produced and then participate in an apparent oxygen transposition in the cascade reaction ( Fig. 3b ) [38] , [39] . 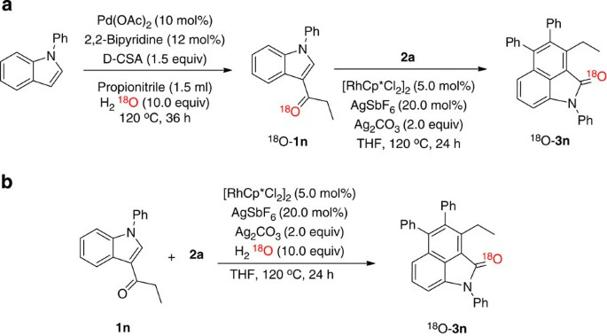Figure 3: Labelling experiments involving18O. (a) The annulation of18O-labelled 1-(1-phenyl-1H-indol-3-yl)propan-1-one (18O-1n) with diphenylacetylene2a. For high-resolution mass spectrometry (HRMS) spectrum of18O-1n, seeSupplementary Fig. 44. For HRMS spectrum of18O-3nobtained from18O-1n, seeSupplementary Fig. 45. (b) The annulation of 1-(1-phenyl-1H-indol-3-yl)propan-1-one (1n) with diphenylacetylene2ain the presence of extra18O-labelled H2O. For HRMS spectrum of18O-3n, seeSupplementary Fig. 46. D-CSA, D-(+)-camphorsulfonic acid. Figure 3: Labelling experiments involving 18 O. ( a ) The annulation of 18 O-labelled 1-(1-phenyl-1 H -indol-3-yl)propan-1-one ( 18 O- 1n ) with diphenylacetylene 2a . For high-resolution mass spectrometry (HRMS) spectrum of 18 O- 1n , see Supplementary Fig. 44 . For HRMS spectrum of 18 O- 3n obtained from 18 O- 1n , see Supplementary Fig. 45 . ( b ) The annulation of 1-(1-phenyl-1 H -indol-3-yl)propan-1-one ( 1n ) with diphenylacetylene 2a in the presence of extra 18 O-labelled H 2 O. For HRMS spectrum of 18 O- 3n , see Supplementary Fig. 46 . D-CSA, D-(+)-camphorsulfonic acid. Full size image On the basis of these above observations, a tentative mechanism of this transformation was proposed to involve the aromatic C4–H activation/cyclization/aromatization via dehydration/nucleophilic addition/oxidation cascade pathway ( Fig. 4 ). We hypothesized that the first step of the catalytic cycle was the formation of the highly electrophilic [Rh(III)Cp*] species A in situ generated from the reaction of [RhCp*Cl 2 ] 2 with AgSbF 6 . Subsequently, the Rh-catalyzed carbonyl-directed regioselective aromatic C4–H activation produced the six-membered rhodacycle B rather than the five-membered rhodium intermediate via the pyrrole C2–H bond activation. An internal alkyne then regioselectively inserted into the rhodium–carbon bond to give an eight-membered rhodacycle C , followed by an intramolecular insertion of the carbonyl group into the rhodium–alkenyl bond to generate the rhodium alkoxide intermediate D (refs 40 , 41 , 42 , 43 ). Subsequent protonation of D provided the possible alcohol intermediate E (refs 8 , 9 , 10 ) and regenerated the active Rh(III) species. The intermediate E underwent aromatization via dehydration to yield the iminium intermediate F (refs 44 , 45 , 46 , 47 ), followed by nucleophilic attack of water. The resulting intermediate G was reoxidized by Ag(I) to furnish the final product, which fulfilled an apparent oxygen transposition via dehydration–rehydration to forge a new carbonyl bond. 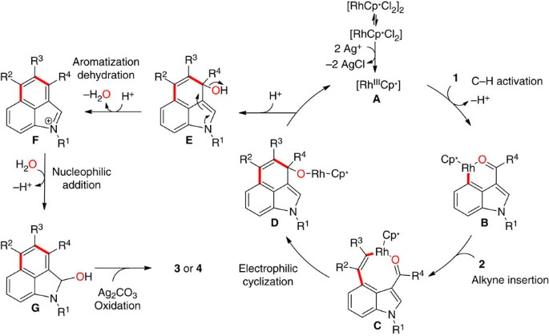Figure 4: Plausible catalytic cycle. The possible mechanism involves the sequential Rh-catalyzed carbonyl-assisted regioselective aromatic C4–H activation/[4+2] cyclization/aromatization via dehydration/nucleophilic addition of water/oxidation. Figure 4: Plausible catalytic cycle. The possible mechanism involves the sequential Rh-catalyzed carbonyl-assisted regioselective aromatic C4–H activation/[4+2] cyclization/aromatization via dehydration/nucleophilic addition of water/oxidation. Full size image To further clarify the proposed mechanism, the electrospray ionization-high-resolution mass spectrometry analysis of the reaction between N -phenyl-indolyl-3-carbaldehyde 1b and diphenylacetylene 2a was performed to capture the possible alcohol intermediate. Fortunately, a peak at m/z 400.1707 appeared, which was in accordance with the intermediate E (R 1 , R 2 , R 3 =Phenyl; R 4 =H) ([M+H] + , MW 400.1701) illustrated in Fig. 4 ( Supplementary Fig. 49 and Supplementary Methods ). However, attempts to separate the intermediate E from the reaction system failed probably due to the rapid dehydration of E . Subsequently, we tried to use 1-(2-methyl-1-phenyl-1 H -indol-3-yl)propan-1-one 1u with a methyl substituent at the indole C2-position as a reaction substrate to isolate the 3-ethyl-2-methyl-1,4,5-triphenyl-1,2-dihydrobenzo[ cd ]indol-2-ol intermediate 5 ( Fig. 5 ). To our surprise, 1u did give rise to the same benzo-fused oxindole product 3n as that of the 2-unsubstituted 1-(1-phenyl-1 H -indol-3-yl)propan-1-one 1n . We assumed that one of the hydrogen atoms of the methyl group at the C2-position might undergo intramolecular dehydration to form the intermediate 6 (refs 9 , 10 ), followed by the oxidation of the terminal alkenyl group to furnish the benzo-fused oxindole 3n in the presence of an excess amount of silver salt [48] . These unexpected observations also well-demonstrated the proposed mechanistic pathway involving the formation of the alcohol intermediate G illustrated in Fig. 4 . 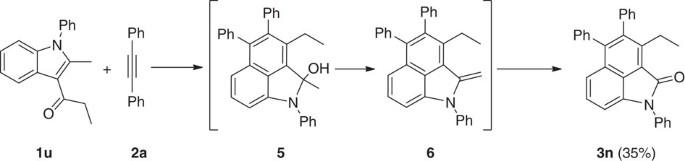Figure 5: The coupling of 1-(2-methyl-1-phenyl-1H-indol-3-yl)propan-1-one 1u with diphenyl acetylene 2a. Reaction conditions:2a(0.25 mmol),1u(2.0 equiv.), [Cp*RhCl2]2(5.0 mol%), AgSbF6(20.0 mol%), Ag2CO3(2.0 equiv.), H2O (2.5 mmol) and THF (2.0 ml) under N2at 120 °C for 24 h. Figure 5: The coupling of 1-(2-methyl-1-phenyl-1 H -indol-3-yl)propan-1-one 1u with diphenyl acetylene 2a. Reaction conditions: 2a (0.25 mmol), 1u (2.0 equiv. ), [Cp*RhCl 2 ] 2 (5.0 mol%), AgSbF 6 (20.0 mol%), Ag 2 CO 3 (2.0 equiv. ), H 2 O (2.5 mmol) and THF (2.0 ml) under N 2 at 120 °C for 24 h. Full size image Improvement of the reactivity and the scope of reaction On the basis of the proposed mechanism, we re-examined the reactivity of indolyl ketones with alkynes by the addition of extra water into the reaction system. As expected, the yields of benzo-fused oxindoles were improved significantly. The yield of 1-(1-phenyl-1 H -indol-3-yl)propan-1-one 1n with diphenyl acetylene 2a was increased from 30 to 61% in the presence of 10.0 equiv. of H 2 O (Comparing 3n in Table 3 with 3n in Table 1 ). As shown in Table 3 , the cascade reaction also exhibited a relatively wide scope of substrates including both indolyl ketones and alkynes. It is worthy to note that unsymmetrical aryl alkyl alkyne could smoothly undergo the regioselective annulation to afford benzo-fused oxindole ( Table 3 , 3t ). In addition, when indolyl aldehydes were used as the substrate, the yields of benzo-fused oxindoles could be increased by ∼ 5%. Table 3 The reaction of indolyl ketones with alkynes. Full size table Synthesis of priolines Priolines, a type of alkaloid, are isolated from the roots of Salvia prionitis [25] . To further elucidate the usefulness of our methodology, the concise synthesis of priolines was performed in four steps starting from7-benzyloxy-6-isopropylindole 7 (ref. 49 ) (For 11a , 21.5% total yield; 11b , 15.3% total yield; 11c , 7.6% total yield; Fig. 6 ). First, compound 7 reacted with benzyl bromide furnished the N -benzyl indole 8 in 84% yield. Subsequently, the acylation at the indole C3-position afforded the crucial intermediate 3-acylated indole 9 in 67% yield by taking advantage of our previously reported method [50] . Indolyl ketone 9 next underwent a regioselective carbon–hydrogen activation/cyclization to give the N - and O -protected priolines 10 . Finally, debenzylation of 10 with trifluoroacetic acid and anisole gave rise to the targeted compounds 11 . 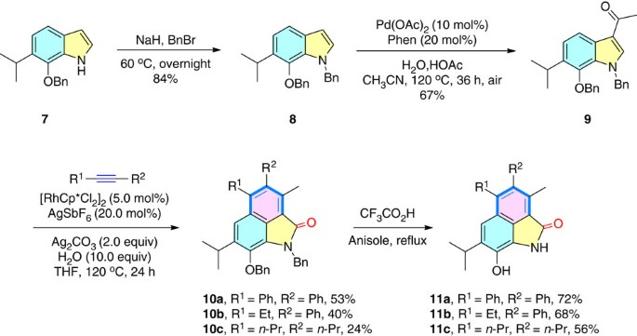Figure 6: Synthesis of priolines 11a–11c. The current tandem reaction was used to construct the key benzo-fused oxindole scaffolds10a–10cin the synthesis of a type of alkaloid isolated from the roots ofSalvia prionitis. Phen, 1,10-phenanthroline. Figure 6: Synthesis of priolines 11a–11c. The current tandem reaction was used to construct the key benzo-fused oxindole scaffolds 10a – 10c in the synthesis of a type of alkaloid isolated from the roots of Salvia prionitis . Phen, 1,10-phenanthroline. Full size image An unprecedented rhodium-catalyzed regioselective carbon–hydrogen activation/cyclization has been disclosed to synthesize benzo-fused oxindoles from easily available indolyl-3-aldehydes or ketones and alkynes, which involves the sequential Rh-catalyzed carbonyl-assisted regioselective aromatic C4–H activation/[4+2] cyclization/aromatization via dehydration/nucleophilic addition of water/oxidation. On the basis of a primary mechanistic investigation, it is found that the addition of extra water can significantly improve the reactivity of indolyl-3-ketones. The catalytic reaction exhibits a high regioselectivity with unsymmetrical alkynes. In addition, the regioselective carbon–hydrogen activation/cyclization has been utilized as the key step for the concise synthesis of priolines. We anticipate that this rhodium-mediated apparent oxygen transposition via dehydration–rehydration would provide us an inspiration for the development of novel and innovative transformations involving a rhodium alkoxide intermediate. This unexpected finding would be useful in the synthesis of natural products and a detailed mechanistic investigation is ongoing in our group. General For 1 H and 13 C NMR analysis of the compounds in this article, see Supplementary Figs 1–41 . General procedure for the reaction of indolyl aldehydes A flame-dried Schlenk tube with a magnetic stir bar was charged with [Cp*RhCl 2 ] 2 (5.4 mg, 8.75 μmol, 3.5 mol%), alkyne (0.25 mmol, 1.0 equiv. ), indolyl aldehyde (0.5 mmol, 2.0 equiv. ), AgSbF 6 (12.0 mg, 0.035 mmol, 14 mol%), Ag 2 CO 3 (82.7 mg, 0.3 mmol, 1.2 equiv.) and THF (3.0 ml) under N 2 . The tube was sealed with a teflon-coated screw cap and the reaction solution was heated at 120 °C for 24 h. The mixture was then cooled to ambient temperature, diluted with 10 ml of CH 2 Cl 2 , filtered through a celite pad and washed with 10–20 ml of CH 2 Cl 2 . The combined organic phases were concentrated and the residue was purified by column chromatography on neutral alumina or silica gel to provide the desired product. General procedure for the reaction of indolyl ketones A flame-dried Schlenk tube with a magnetic stir bar was charged with [Cp*RhCl 2 ] 2 (7.8 mg, 12.5 μmol, 5.0 mol%), alkyne (0.25 mmol, 1.0 equiv. ), indolyl ketone (0.5 mmol, 2.0 equiv. ), AgSbF 6 (17.2 mg, 0.05 mmol, 20 mol%), Ag 2 CO 3 (137.9 mg, 0.5 mmol, 2.0 equiv. ), H 2 O (45 μl, 2.5 mmol, 10.0 equiv.) and THF (2.0 ml) under N 2 . The tube was sealed with a teflon-coated screw cap and the reaction solution was heated at 120 °C for 24 h. The mixture was then cooled to ambient temperature, diluted with 10 ml of CH 2 Cl 2 , filtered through a celite pad and washed with 10–20 ml of CH 2 Cl 2 . The combined organic phases were concentrated and the residue was purified by column chromatography on silica gel to provide the desired product. How to cite this article: Liu, X. et al. Unexpected regioselective carbon–hydrogen bond activation/cyclization of indolyl aldehydes or ketones with alkynes to benzo-fused oxindoles. Nat. Commun. 5:5030 doi: 10.1038/ncomms6030 (2014). Accession codes: The X-ray crystallographic coordinates for structures reported in this article have been deposited at the Cambridge Crystallographic Data Centre (CCDC), under deposition number CCDC 979092 ( 3a ) and CCDC 979091 ( 3n ). These data can be obtained free of charge from The Cambridge Crystallographic Data Centre via www.ccdc.cam.ac.uk/data_request/cif